Lipid-dependent gating of a voltage-gated potassium channel Recent studies hypothesized that phospholipids stabilize two voltage-sensing arginine residues of certain voltage-gated potassium channels in activated conformations. It remains unclear how lipids directly affect these channels. Here, by examining the conformations of the KvAP in different lipids, we showed that without voltage change, the voltage-sensor domains switched from the activated to the resting state when their surrounding lipids were changed from phospholipids to nonphospholipids. Such lipid-determined conformational change was coupled to the ion-conducting pore, suggesting that parallel to voltage gating, the channel is gated by its annular lipids. Our measurements recognized that the energetic cost of lipid-dependent gating approaches that of voltage gating, but kinetically it appears much slower. Our data support that a channel and its surrounding lipids together constitute a functional unit, and natural nonphospholipids such as cholesterol should exert strong effects on voltage-gated channels. Our first observation of lipid-dependent gating may have general implications to other membrane proteins. Voltage-gated ion channels have essential roles in many physiological activities [1] . Biophysical mechanisms underlying their function have been studied extensively, but fundamental questions remain open regarding the voltage-driven conformational changes of the voltage-sensing domains (VSDs) in these channels [2] , [3] , [4] , [5] , [6] . Generally, the VSDs switch from a 'down' (also called the resting, deactivated or closed state) to an 'up' conformation (alternatively named the activated or open state) when the transmembrane potential is depolarized [4] , [5] , [6] , [7] , [8] , [9] . Four highly conserved positively charged residues in the fourth transmembrane segment (S4) of the VSD contribute a major fraction of the 'gating charge', ~13 elementary units per Shaker -like channel [10] , [11] , [12] , [13] . The VSD movement and its electro-mechanical coupling to the ion-conducting pore are the two intrinsic characteristics of voltage-dependent gating. Several distinct models for the VSD movement have arisen from past studies [2] , [3] , [4] , [5] , [14] , [15] , [16] , [17] , [18] , [19] , [20] , [21] , [22] , [23] , [24] . The discrepancies among these models in part resulted from differences in experimental systems—functional studies of channels in membranes versus structural investigations of the proteins in detergents, and the lack of good understanding of how lipids directly influence the VSDs. Protein–lipid interaction has been shown to be important for many membrane proteins [25] . For some proteins, lipids even serve as a topogenetic determinant [26] . In cell membranes, proteins may reside in specialized microdomains that have specific lipid composition and can modulate protein function [27] , [28] , [29] , [30] . Some mammalian voltage-gated channels were detected in membrane microdomains even though the functional effects of such localization remain poorly understood, largely due to technical difficulties in studying channels exclusively in these microdomains [31] , [32] . Recently lipid phosphodiesters and enzymatic modification of sphingomyelin head groups were showed to exert strong influence on certain voltage-gated potassium (Kv) channels [33] , [34] , [35] . It was hypothesized that the phosphodiester groups stabilize the lipid-facing voltage-sensing residues in the 'up' conformation. No evidence exists for direct interactions of phosphodiesters with the S4-gating arginines in membranes, and the mechanistic understanding of lipid-VSD interaction is rather vague. The experiments presented below are aimed at testing the current reigning hypothesis and investigating the effect of lipid–VSD interaction on the conformational change of the VSDs. The intrinsic heterogeneity of native cell membranes makes it difficult to dissect the lipid effects on voltage-gated ion channels. We instead used as a model system the KvAP channel from Aeropyrum pernix in artificial membranes, either black lipid membranes or lipid vesicles with well-defined lipid composition, and developed conformation-specific assays to assess the conformations of the VSDs and the channel pore. Our results showed that switching a KvAP channel from membranes of nonphospholipids to phospholipids shifted the VSDs between two gating conformations and directly gated the ion-conducting pore. Our analysis suggested that the phosphate–arginine interaction is not required for voltage-dependent gating, but instead the lipids immediately around the VSDs contribute to the lipid-dependent gating. Our working hypothesis predicts that lipid components such as cholesterol should have strong effects on channel function, and our experiments confirmed the expected cholesterol effect. Together our results demonstrate that the annular lipids around the VSDs constitute a new gating modality for a Kv channel. A conformation-specific ligand for the KvAP VSD To assess lipid effects on the VSD, we developed assays to detect its specific conformations. Our first assay used a recombinant immunoglobulin domain (Fv) that binds to the tip of the KvAP voltage-sensor paddle [36] , and inhibits the channel activity. Fv-binding to channels in a phospholipid bilayer (3:1 1-palmitoyl-2-oleoyl- sn -3-glycero-phosphoethanolamine (POPE)/1-palmitoyl-2-oleoyl- sn-3 -glycero-phosphoglycerol (POPG), PE/PG hereafter; Supplementary Fig. S1 ) exhibited strong voltage-dependence ( Fig. 1a and Supplementary Note 1 ). From −90 to −60 mV, the VSD switched from an Fv-inaccessible state to an accessible one ( Fig. 1b ). Such a transition has an apparent gating charge ( Zδ ) of 5.0 e 0 , and a mid-point potential V 1/2 of −70.3 mV, which is ~35 mV left-shifted from a typical conductance-voltage curve of the KvAP in PE/PG membranes. The voltage-dependent Fv inhibition closely reflects the voltage dependence of the VSD movement. Comparison of our measurements ( Fig. 1b ) with those from the Shaker channel [37] , [38] indicates that all four KvAP VSDs need to switch to the 'up' conformation before its pore domain gains substantial open probability. 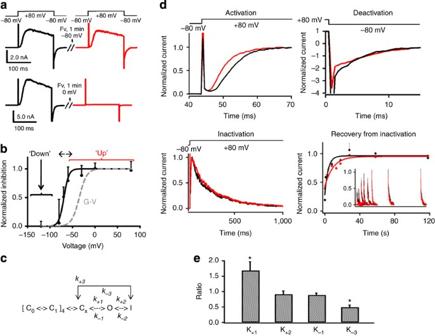Figure 1: An up-conformation-specific binder for KvAP VSDs. (a) Voltage-dependence of Fv-Binding. Fv (1.0 μg ml−1) was perfused to thecisside of a stable bilayer held at a test potential for 1 min. After the treatment, the membrane was returned to −80 mV for 2 min before next test pulse. Current traces before (black) and after (red) Fv treatment at −80 mV and 0 mV are presented. (b) Normalized inhibition plotted against testing potentials (black dots, mean±s.d.,n=4). Boltzmann fitting (black line) yieldedV1/2=−70.3±1.1 mV,Zδ=5.0±0.97. The grey dashed line is a typical G–V curve of KvAP withV1/2=−35 mV,Zδ=3.5. (c) A gating scheme.C1,Cx,O,Iare Fv-accessible. At depolarization,k−2,k+3are negligibly small. (d) Top two panels show typical traces of activation (+80 mV) and deactivation (–80 mV) before (black) and after (red) Fv treatment. Bottom left is the inactivation at +80 mV without (black) and with (red) Fv. Bottom right shows the recovery from inactivation at −80 mV before (black) and after (red) Fv treatment by using a paired-pulse protocol. Inset showed two trains of normalized traces (red +Fv, black control) elicited by the second of the paired pulses plotted against specific intervals between paired pulses. (e) Fv-induced changes in kinetic rates (P<0.036 forK+1,P<0.016 forK−3; error bars represent s.d.,n=4).Ki=ki,Fv/ki,no Fv, i=±1,+2,–3 (Supplementary Note S2,K+1=1.68+0.29,K+2=0.91+0.11,K−1=0.89+0.07 andK−3=0.49+0.074, mean±s.d.,n=4). When measuredk−3andk−1are used at depolarization voltages, [FvI]/[FvC] ~3.5-folds of [I]/[C]. Figure 1: An up-conformation-specific binder for KvAP VSDs. ( a ) Voltage-dependence of Fv-Binding. Fv (1.0 μg ml −1 ) was perfused to the cis side of a stable bilayer held at a test potential for 1 min. After the treatment, the membrane was returned to −80 mV for 2 min before next test pulse. Current traces before (black) and after (red) Fv treatment at −80 mV and 0 mV are presented. ( b ) Normalized inhibition plotted against testing potentials (black dots, mean±s.d., n =4). Boltzmann fitting (black line) yielded V 1/2 =−70.3±1.1 mV, Zδ =5.0±0.97. The grey dashed line is a typical G–V curve of KvAP with V 1/2 =−35 mV, Zδ= 3.5. ( c ) A gating scheme. C 1 , C x , O , I are Fv-accessible. At depolarization, k −2 , k +3 are negligibly small. ( d ) Top two panels show typical traces of activation (+80 mV) and deactivation (–80 mV) before (black) and after (red) Fv treatment. Bottom left is the inactivation at +80 mV without (black) and with (red) Fv. Bottom right shows the recovery from inactivation at −80 mV before (black) and after (red) Fv treatment by using a paired-pulse protocol. Inset showed two trains of normalized traces (red +Fv, black control) elicited by the second of the paired pulses plotted against specific intervals between paired pulses. ( e ) Fv-induced changes in kinetic rates ( P <0.036 for K +1 , P <0.016 for K −3 ; error bars represent s.d., n =4). K i = k i,Fv / k i,no Fv , i= ±1,+2,–3 ( Supplementary Note S2 , K +1 =1.68+0.29, K +2 =0.91+0.11, K −1 =0.89+0.07 and K −3 =0.49+0.074, mean±s.d., n =4). When measured k −3 and k −1 are used at depolarization voltages, [FvI]/[FvC] ~3.5-folds of [I]/[C]. Full size image On the basis of a general gating scheme [37] ( Fig. 1c ), Fv should recognize multiple gating states (all except C 0 ). Fv-binding could keep the VSDs 'up', and then either inactivate the channel pore domain or stabilize the channel in intermediate closed states ( C 1 or C x ). Measuring the gating kinetics of KvAP ( Fig. 1d and Supplementary Note 2 ) showed that at low concentrations Fv-binding accelerated the concerted opening step ( C x → O , k +1 ) and slowed down the recovery from inactivation ( k −3 ), but it did not alter significantly the deactivation ( k −1 ) and inactivation ( k +2 , Fig. 1e ). The net result is that Fv-binding favours the inactivated state. Further analysis of the time-dependent Fv effect yielded its elementary ON-rate ( k on ~1.2×10 5 s −1 M −1 ), EC50 (0.65 μg ml −1 , ~30 nM) and slow washout ( k off ~1/20 min −1 , Supplementary Fig. S2 and Supplementary Note 3 ). The estimated Fv affinity ( k D ) is ~10 nM, close to EC50 . If corrected for the actual duration of the Fv-accessible states, the affinity would be ~10–20 pM, which agrees with the fact that good Fab fragments exhibit picomolar affinity and channels in lipid bilayers are spatially restricted with three fewer degrees of freedom and thus more efficient for Fv-binding. The linear relation between apparent ON-rates and [Fv] indicates that either Fv-binding on one VSD of a channel is enough to inhibit its ion-conducting activity, or binding of one Fv is rate limiting. Fv therefore effectively recognizes the VSDs in the 'up' conformation. VSDs in nonphospholipids apparently reside in a 'down' conformation The voltage-dependent Fv inhibition allows us to quantify indirectly the VSD movement in membranes containing a fraction of nonphospholipids (lipids without phosphodiesters; 1,2-dioleoyl-3-trimethylammonium-propane (DOTAP) and 1,2-dioleoyl- sn -glycero-3-succinate (DOGS) as examples, Supplementary Fig. S1 ). Low %DOTAP and %DOGS both rendered the voltage dependence of Fv-induced inhibition slightly right-shifted and shallower ( Fig. 2a ), meaning that they increase the energetic cost for the VSDs to switch from 'down' to 'up'. 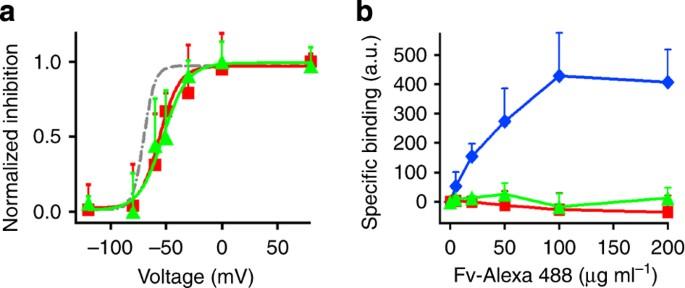Figure 2: Nonphospholipids render it difficult for the VSD to switch to the 'up' conformation. (a) Voltage-dependent Fv inhibition of KvAP activity was measured in PE/PG bilayers containing low DOTAP (<10% in weight ratio; red squares, s.d.;n=3) or DOGS (<10% by weight; green triangles, s.d.;n=3). Fitting with a Boltzmann function gaveV1/2=−55.3±2.1 mV,Zδ =2.5±0.66 (red line), andV1/2=−52.8±2.8 mV,Zδ=2.6±0.62 (green line). As a control, the black curve inFigure 1bis shown as a dashed grey line. (b) Binding of Fv-Alexa 488 to reconstituted KvAP in vesicles of different lipids was measured (blue diamonds for PE/PG, red squares for DOTAP and green triangles for DOGS; error bars represent s.d.;n=4–5). Figure 2: Nonphospholipids render it difficult for the VSD to switch to the 'up' conformation. ( a ) Voltage-dependent Fv inhibition of KvAP activity was measured in PE/PG bilayers containing low DOTAP (<10% in weight ratio; red squares, s.d. ; n =3) or DOGS (<10% by weight; green triangles, s.d. ; n =3). Fitting with a Boltzmann function gave V 1/2 =−55.3±2.1 mV, Zδ = 2.5±0.66 (red line), and V 1/2 =−52.8±2.8 mV, Zδ =2.6±0.62 (green line). As a control, the black curve in Figure 1b is shown as a dashed grey line. ( b ) Binding of Fv-Alexa 488 to reconstituted KvAP in vesicles of different lipids was measured (blue diamonds for PE/PG, red squares for DOTAP and green triangles for DOGS; error bars represent s.d. ; n =4–5). Full size image To quantify the VSD conformation in pure DOTAP or DOGS membranes, a Fv-Alexa 488 was produced for an 'up'-conformation specific binding assay ( Supplementary Fig. S3a and b ). As expected, Fv-Alexa 488 binds avidly to KvAP in PE/PG membranes. But to our surprise, it failed to recognize channels in DOTAP or DOGS ( Fig. 2b ). Our floatation experiments showed that even though their VSDs were inaccessible to Fv, almost all channels were incorporated in DOTAP or DOGS vesicles ( Supplementary Fig. S4 ). When channels in DOTAP or DOGS were fused into phospholipid bilayers, they regained their activity, suggesting that they were not irreversibly denatured or trapped in nonnative states [33] . To test whether the KvAP channel pore was properly folded, a charybdotoxin (CTX)-Alexa 488 conjugate ( Fig. 3a,b ) was prepared to check the tetrameric state of the KvAP protein in vesicles ( Fig. 3c,d ). Because of the high concentration of unlabelled CTX used in control samples, the CTX-Alexa 488 was limited to 5.0 μM here. The lower CTX affinity to channels in negatively charged DOGS membranes might have resulted from the nonphospholipids occupying the phospholipid-binding sites that are similar to those seen in the structures of KcSA and Kv1.2/2.1 chimera [22] , [39] . Nevertheless, the observed significant CTX-binding suggests that channel pores in DOGS are tetrameric, the same as in DOTAP [40] ( Fig. 3d ). These data led us to question the possibility that VSDs in DOTAP or DOGS might be kept 'down'. 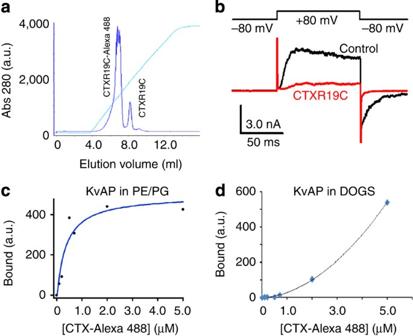Figure 3: Channels in DOGS vesicles appear folded properly. (a) Elution of CTX-R19C-Alexa 488 from a Resource S FPLC column. The ionic gradient (cyan trace) of NaCl varied from 30 to 500 mM. The conjugate eluted at ~150 mM NaCl with a noisy peak tip due to detector saturation. (b) Recombinant CTXR19C was active on the KvAP channels in lipid bilayers. In all, 200 nM CTXR19C was added to the extracellular side of the bilayer, which inhibited almost all channel activity after 10 min (red trace against the black control). (c) CTXR19C-Alexa 488 binding to the KvAP channels in PE/PG vesicles. Vesicles were incubated with CTX-Alexa 488 in a small volume, and then pelleted down at 250,000gfor 45 min. The pellet was resuspended in a DM buffer for fluorescence measurement. For each data point (black dots), a control sample with 100 μM CTX was prepared to measure nonspecific binding, and specific binding was plotted as a function of the CTX-Alexa 488 concentration. Fitting of the data (blue line) with a Michaelis–Menten equation yielded akDof 350 nM, lower than unconjugated toxin. (d) Binding of CTX-Alexa 488 to the KvAP channels in DOGS vesicles (blue diamonds with a black line from polynomial fitting). Even though the DOGS membranes decrease the affinity of KvAP to CTX-Alexa 488 (kD> 2.0 μM), there was still high specific CTX-binding at 2.0 and 5.0 μM of CTX-Alexa 488. Figure 3: Channels in DOGS vesicles appear folded properly. ( a ) Elution of CTX-R19C-Alexa 488 from a Resource S FPLC column. The ionic gradient (cyan trace) of NaCl varied from 30 to 500 mM. The conjugate eluted at ~150 mM NaCl with a noisy peak tip due to detector saturation. ( b ) Recombinant CTXR19C was active on the KvAP channels in lipid bilayers. In all, 200 nM CTXR19C was added to the extracellular side of the bilayer, which inhibited almost all channel activity after 10 min (red trace against the black control). ( c ) CTXR19C-Alexa 488 binding to the KvAP channels in PE/PG vesicles. Vesicles were incubated with CTX-Alexa 488 in a small volume, and then pelleted down at 250,000 g for 45 min. The pellet was resuspended in a DM buffer for fluorescence measurement. For each data point (black dots), a control sample with 100 μM CTX was prepared to measure nonspecific binding, and specific binding was plotted as a function of the CTX-Alexa 488 concentration. Fitting of the data (blue line) with a Michaelis–Menten equation yielded a k D of 350 nM, lower than unconjugated toxin. ( d ) Binding of CTX-Alexa 488 to the KvAP channels in DOGS vesicles (blue diamonds with a black line from polynomial fitting). Even though the DOGS membranes decrease the affinity of KvAP to CTX-Alexa 488 ( k D > 2.0 μM), there was still high specific CTX-binding at 2.0 and 5.0 μM of CTX-Alexa 488. Full size image To verify such a 'down' conformation, we tested cysteine accessibility in two specific sites of the VSD—L125 and F124. Similar to an equivalent site in the Shaker channel, L125C is accessible from the intracellular side only when the VSDs are 'down' [2] , [41] . KvAPΔ36 is a functional cys-less mutant lacking the carboxy terminal 36 residues, and was used to introduce single-cysteine residues. Truncation removed the native cys247 and eliminated crosslinked dimers seen in the wild-type channels ( Supplementary Fig. S5 ). Methoxy-poly-(ethylene glycol)-5000-succinamidoethyl methane-thiosulfonate (MTSPEG5k) was introduced to modify the introduced single-cysteine residues. PEGylation (PEG-ed in Fig. 4a,b ) caused a 5.0-kDa shift to the protein bands in nonreducing SDS polyacrylamide gel electrophoresis (SDS–PAGE; gel-shift assay). KvAPΔ36L125C in PE/PG was inaccessible, but in DOTAP, the cysteine was modified ( Fig. 4a ). Because of random channel orientation in vesicles and membrane impermeability of MTSPEG5k, the expected PEGylation level of L125C is ~50%, close to our observation. As a control, we exploited our observation that a channel/Fv complex reconstituted in DOTAP retained its Fv, probably because four high-affinity Fv molecules cooperatively kept all VSDs 'up'. The KvAPΔ36L125C/Fv complexes in PE/PG or DOTAP were thus not PEGylated ( Fig. 4a ). 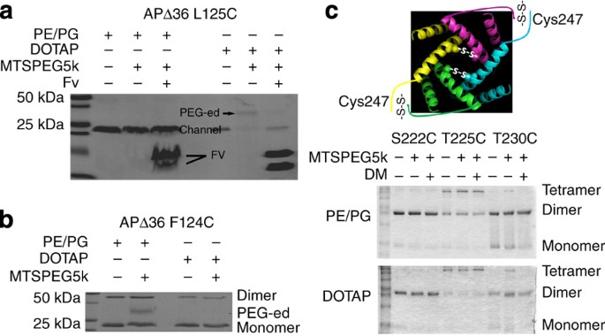Figure 4: Nonphospholipids favour KvAP VSDs in the 'down' conformation. (a) Gel-shift assay of KvAPΔ36L125C. Vesicles were reduced with 5.0 mM DTT or 2.0 mM TCEP (tris (2-carboxyethyl) phosphine), pelleted to remove DTT (or TCEP), reacted with 2.0 mM MTSPEG5k for 30 min at room temperature. Vesicles with Fv-bound channels were control. MTSPEG5k conjugation shifted the channel band by ~5 kDa (black arrow). Before channels in DOTAP were mixed with SDS-buffer, 20 mM decyl-maltoside (DM) was added to rescue 20–50% of the protein, which made the Coomassie blue-stained bands weaker than those from other vesicles. (b) Similar toa, reconstituted APΔ36F124C was tested for accessibility in PE/PG and DOTAP. (c) Tetramerization assay of full-length KvAP-T225C. Top ribbon diagram highlights the intracellular surface of the KvAP open-pore structure (PDB code 2A0L, generated in PYMOL; DeLano Scientific). Four pairs of disulphide bonds (–S–S–) in a crosslinked tetrameric pore are showed schematically. Side chains of four T225 residues are shown as spherical balls. At the bottom, reconstituted channels in PE/PG and DOTAP were compared in nonreducing SDS–PAGE. Vesicles were reduced with 5.0 mM DTT for 30 min at 4 °C, pelleted at 200,000gfor 45 min, washed and resuspended in a buffer containing 5.0 mM GSSG. After 30-min incubation at room temperature, the vesicles were assayed in 15% nonreducing SDS–PAGE. Most T225C mutants in DOTAP ran as crosslinked tetramers, whereas in PE/PG, only 40––50% channels did. Addition of MTSPEG5k or 20 mM DM after the GSSG treatment did not make a difference. Repeated experiments of T225C always showed more than 85% crosslinked tetramers in DOTAP and only ~50% in PE/PG. Figure 4: Nonphospholipids favour KvAP VSDs in the 'down' conformation. ( a ) Gel-shift assay of KvAPΔ36L125C. Vesicles were reduced with 5.0 mM DTT or 2.0 mM TCEP (tris (2-carboxyethyl) phosphine), pelleted to remove DTT (or TCEP), reacted with 2.0 mM MTSPEG5k for 30 min at room temperature. Vesicles with Fv-bound channels were control. MTSPEG5k conjugation shifted the channel band by ~5 kDa (black arrow). Before channels in DOTAP were mixed with SDS-buffer, 20 mM decyl-maltoside (DM) was added to rescue 20–50% of the protein, which made the Coomassie blue-stained bands weaker than those from other vesicles. ( b ) Similar to a , reconstituted APΔ36F124C was tested for accessibility in PE/PG and DOTAP. ( c ) Tetramerization assay of full-length KvAP-T225C. Top ribbon diagram highlights the intracellular surface of the KvAP open-pore structure (PDB code 2A0L, generated in PYMOL; DeLano Scientific). Four pairs of disulphide bonds (–S–S–) in a crosslinked tetrameric pore are showed schematically. Side chains of four T225 residues are shown as spherical balls. At the bottom, reconstituted channels in PE/PG and DOTAP were compared in nonreducing SDS–PAGE. Vesicles were reduced with 5.0 mM DTT for 30 min at 4 °C, pelleted at 200,000 g for 45 min, washed and resuspended in a buffer containing 5.0 mM GSSG. After 30-min incubation at room temperature, the vesicles were assayed in 15% nonreducing SDS–PAGE. Most T225C mutants in DOTAP ran as crosslinked tetramers, whereas in PE/PG, only 40––50% channels did. Addition of MTSPEG5k or 20 mM DM after the GSSG treatment did not make a difference. Repeated experiments of T225C always showed more than 85% crosslinked tetramers in DOTAP and only ~50% in PE/PG. Full size image Residue F124C showed a state-dependent accessibility opposite to that of L125C in lipid bilayers [2] . KvAPΔ36F124C in PE/PG was reactive to MTSPEG5k, but in DOTAP it was inaccessible ( Fig. 4b ). Because SDS-binding to DOTAP led to some protein precipitation, the KvAP bands from DOTAP vesicles were fainter in SDS–PAGE gels. But it did not affect the determination of cysteine accessibility. Similarly, the observed crosslinked F124C dimers (through disulphides) did not compromise our experiments either. Together our observations in L125C and F124C evidenced that the VSDs in DOTAP are likely in a 'down' conformation. The 'down' conformation in nonphosplipids appears native We next examined the nature of the nonphospholipid-determined 'down' state from three different aspects. When the cysteine accessibility analysis was done at other VSD residues ( Table 1 ), all functional mutants in PE/PG or DOTAP behaved exactly the same as in native 'up' and 'down' conformations in phospholipids [2] , [42] , [43] . These data argue that the VSDs in DOTAP or DOGS do not take the nonnative conformations as seen in the multiple crystal structures of the KvAP [36] , [44] in detergents, but apparently are in the native 'down' state. Table 1 Cys-accessibility of KvAPΔ36 mutants in PE/PG versus in DOTAP. Full size table VSDs in the 'down' conformation in DOTAP are expected to drive the channel pore into its closed state. We developed a tetramerization assay to examine the pore conformation. In the open-pore structure of the full-length KvAP [44] ( Fig. 4c , top panel), T225 residues from neighbouring subunits are the closest to each other ( C α –C α distance of 12 Å) at the intracellular gate. They could become even closer when the pore is closed, and if at right orientations, allow disulphide formation. Together with Cys247, T225C disulphides would lead to crosslinked tetramers. S222C and T230C, both are approximately one helical turn away from T225, served as negative controls, and were mostly crosslinked dimers in both PE/PG and DOTAP (cys247 disulphides, Fig. 4c and Supplementary Fig. S5 ). In contrast, 40–50% of the KvAP–T225C mutants in PE/PG were tetrameric in nonreducing SDS–PAGE. In DOTAP, this ratio went up to ~90%, indicating that the channel pore is largely closed in DOTAP, which agrees well with the VSDs being 'down' and coupled to the pore domain. If the 'down' conformation in DOTAP or DOGS is native, a specific ligand recognizing this conformation should bind the VSDs under hyperpolarization in phospholipids. From a phage-displayed peptide library, four positive clones were isolated against the KvAP channels in DOTAP and DOGS ( Supplementary Fig. S6 ). Among these four we showed the results for one (referred to as φ D hereafter). Phage φ D inhibited the channel activity from the intracellular side with EC 50 ~125 nM ( Fig. 5a ). With five copies of the peptide, its dose-dependent effect follows almost a linear relation ( Supplementary Note 4 ), suggesting that one phage is probably enough to inhibit one channel. 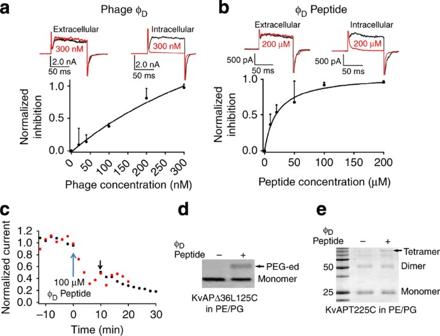Figure 5: A 'down' conformation-specific ligand for KvAP in phospholipids. (a) Phage φDinhibits channels in PE/PG. Top shows current traces with 300 nM phages on either side of the bilayer (black and red traces recorded before and 20 min after phage addition, respectively). Bottom is the dose-dependence for intracellular phage (black dots, s.d.;n=3). The continuous line is a polynomial fit (Supplementary Note S4). (b) Synthetic φDpeptide (GNHAEIYSNHHMMSHVGGGR) inhibits KvAP. Top traces represent typical results for 200 μM peptide on either side of the bilayer (black and red traces recorded before and 20 min after peptide addition, respectively). The bottom shows the normalized inhibition (I) versus peptide concentration (black dots, s.d.;n=3; black line from a fitting withI=Imax/(1+kD/[peptide]),kD=21.2±3.5 μM). (c) φDPeptide binds to channels in resting state. Peptides at a concentration of 100 μM were added to the intracellular side at time 0. Two procedures were compared. One was that test pulses were delivered every 2 min (red dots). The other was that after the addition of the peptide, the membrane was held at −80 mV for 10 min before the delivery of next test pulse (black dots). The black arrow marks the first response after 10 min silence. (d) φDpeptide makes KvAPΔ36L125C accessible in PE/PG. In the presence (+) or absence (+) of 100 μM peptide, channels were reduced, separated from reducing agents, incubated with 1.0 mM MTSPEG5k, quenched with 10 mM iodoacetamide and analysed in 15% nonreducing SDS–PAGE. (e) φDPeptide favoured the closed pore. In presence (+) or absence (−) of 100 μM peptide, full-length KvAP-T225C in PE/PG were reduced, separated from reducing agent and treated with 5.0 mM GSSG peptide for 2–3 min ('blank period') before nonreducing SDS––PAGE. Figure 5: A 'down' conformation-specific ligand for KvAP in phospholipids. ( a ) Phage φ D inhibits channels in PE/PG. Top shows current traces with 300 nM phages on either side of the bilayer (black and red traces recorded before and 20 min after phage addition, respectively). Bottom is the dose-dependence for intracellular phage (black dots, s.d. ; n =3). The continuous line is a polynomial fit ( Supplementary Note S4 ). ( b ) Synthetic φ D peptide (GNHAEIYSNHHMMSHVGGGR) inhibits KvAP. Top traces represent typical results for 200 μM peptide on either side of the bilayer (black and red traces recorded before and 20 min after peptide addition, respectively). The bottom shows the normalized inhibition ( I ) versus peptide concentration (black dots, s.d. ; n =3; black line from a fitting with I=I max /(1 +k D /[peptide]), k D =21.2±3.5 μM). ( c ) φ D Peptide binds to channels in resting state. Peptides at a concentration of 100 μM were added to the intracellular side at time 0. Two procedures were compared. One was that test pulses were delivered every 2 min (red dots). The other was that after the addition of the peptide, the membrane was held at −80 mV for 10 min before the delivery of next test pulse (black dots). The black arrow marks the first response after 10 min silence. ( d ) φ D peptide makes KvAPΔ36L125C accessible in PE/PG. In the presence (+) or absence (+) of 100 μM peptide, channels were reduced, separated from reducing agents, incubated with 1.0 mM MTSPEG5k, quenched with 10 mM iodoacetamide and analysed in 15% nonreducing SDS–PAGE. ( e ) φ D Peptide favoured the closed pore. In presence (+) or absence (−) of 100 μM peptide, full-length KvAP-T225C in PE/PG were reduced, separated from reducing agent and treated with 5.0 mM GSSG peptide for 2–3 min ('blank period') before nonreducing SDS––PAGE. Full size image To confirm that φ D recognizes the VSD in the native 'down' conformation, its peptide was synthesized for our assays. The intracellular peptide inhibited KvAP activity in PE/PG membranes, following a 'single-binding-site' model with k D ~20 μM ( Fig. 5b ). Its lower affinity than the phage was probably due to its decreased copy number. The peptide was effective on KvAP channels in the resting state (−80 mV), VSDs of which were kept in the native 'down' conformation ( Fig. 5c ). In the presence of the peptide, KvAPΔ36-L125C channels in PE/PG became accessible to MTSPEG5k ( Fig. 5d ). The lesser extent of PEGylation in Fig. 5d was probably because the peptide was not as efficient as a DOTAP or DOGS bilayer in maintaining homogeneous 'down' conformation. When the peptide was used in T225C-tetramerization experiments as in Fig. 4c , the crosslinked tetrameric KvAP-T225C in PE/PG vesicles increased from ~50% to 60–70% (close to the expected maximum ~75%; data not shown). This result was not clear-cut. As an alternative, we exploited our observation that the crosslinked KvAPT225C tetramers in PE/PG membranes did not appear during the first several minutes after the channels were reduced and the reducing reagents were removed (called the 'blank period'; control in Fig. 5e ). The φ D peptide promoted a significant fraction of crosslinked tetramers in the 'blank period' (arrow in Fig. 5d ) because it stabilized the channels in the native resting state. Together with the phage data, our observations demonstrated that the nonphospholipid-determined 'down' conformation and the hyperpolarization-induced native 'down' conformation in phospholipids were recognized by the same ligands, and probably are thus very close to each other. Three lines of evidence from very different angles converged to the inevitable conclusion that the 'down' conformation of the VSDs in nonphospholipids matches well the native hyperpolarization-driven 'down' conformation and is tightly coupled to the pore domain. Switching between phospholipids and nonphospholipids therefore gates the channel by changing the conformation of the VSDs, which will be called 'lipid-dependent gating'. Phospholipids as a determinant for lipid-dependent gating The homogeneous lipid-determined conformations made it possible to test the earlier hypothesis that the phosphates stabilize two of the gating Arg residues in the 'up' conformation [6] , [45] . If this hypothesis holds, mutating either one or both of the first two S4 arginine residues into neutral or negatively charged ones would prevent the VSDs from switching 'up'. This is not the case for either KvAP or the Shaker channel [2] , [19] , [23] , [46] , [47] . Our mutants, KvAPΔ36 R117C, R120C and R117H/R120H, were all able to open in phospholipids. Moreover, if stabilizing the arginines in the 'up' conformation were the only critical requirement, removal of both arginines and phosphodiesters should allow the VSDs in nonphospholipids to reach the 'up' conformation. This was not detected in the Fv-Alexa 488-binding assays either ( Fig. 6a,b ), suggesting that the absolute necessity of phosphodiesters for KvAP function [33] did not result from satisfying the first two S4 arginines, but was for switching the whole VSD to its 'up' state. On the other hand, the arginine–phosphate interaction is not required for the VSDs to reach the 'down' conformation because both the wild-type KvAP and its multiple mutants could switch 'down' ( Figs 2 , 4 , 6 ). This conclusion is not surprising because the S4 arginine residues in the 'down' conformation are thought to be less lipid-exposed [2] , [15] , [23] , [48] . 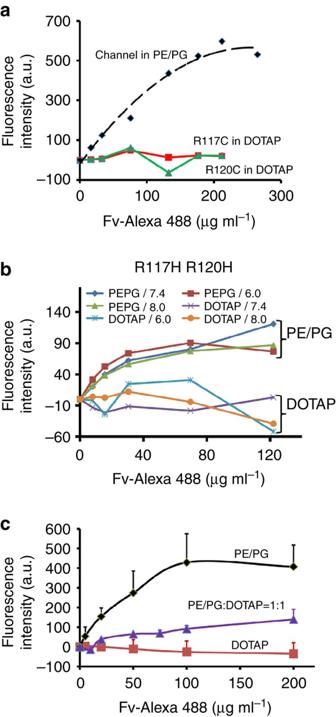Figure 6: Requirement of phosphate groups for the lipid-dependent gating. (a) KvAP R117C (red squares) and R120C (green triangles) in DOTAP membranes do not have specific Fv-binding. As a control, KvAP in PE/PG (black diamonds with a black dashed trend line) shows high specific Fv-binding. (b) KvAP R117H/R120H mutant channels in PE/PG membranes (0.10 mg ml−1protein instead of 0.50 mg ml−1because of the low-expression level of the mutant) have specific Fv-binding at pH 6.0, 7.4 and 8.0, but not in DOTAP membranes at all three pHs. The data at three pH levels showed the reproducibility of the binding assay even at low concentrations of channel protein. (c) In vesicles of 1:1 ratio of PE/PG: DOTAP (purple triangles;n=2, error bars are range of variation) the KvAP channels had only about 25% of the Fv-binding activity as the same quantity of channels in PE/PG (black diamonds,n=5, s.d.). The binding curve of channels in DOTAP (red squares,n=5, s.d.) is shown as a control. Figure 6: Requirement of phosphate groups for the lipid-dependent gating. ( a ) KvAP R117C (red squares) and R120C (green triangles) in DOTAP membranes do not have specific Fv-binding. As a control, KvAP in PE/PG (black diamonds with a black dashed trend line) shows high specific Fv-binding. ( b ) KvAP R117H/R120H mutant channels in PE/PG membranes (0.10 mg ml −1 protein instead of 0.50 mg ml −1 because of the low-expression level of the mutant) have specific Fv-binding at pH 6.0, 7.4 and 8.0, but not in DOTAP membranes at all three pHs. The data at three pH levels showed the reproducibility of the binding assay even at low concentrations of channel protein. ( c ) In vesicles of 1:1 ratio of PE/PG: DOTAP (purple triangles; n =2, error bars are range of variation) the KvAP channels had only about 25% of the Fv-binding activity as the same quantity of channels in PE/PG (black diamonds, n =5, s.d.). The binding curve of channels in DOTAP (red squares, n =5, s.d.) is shown as a control. Full size image What is the chemical nature of the phosphodiester–VSD interaction? If any high-affinity lipid-binding site on the VSDs is dominantly critical [22] , [34] , [35] , 50% of phospholipids (equivalent to ~750 mM by using a 55×20 Å 3 volume for each lipid molecule) in a well-mixed bilayer should saturate such a site, and restore the channel function almost completely. In membranes of 1:1 (weight ratio) phospholipids/DOTAP, the KvAP channels had only ~25% of Fv-binding activity as the same quantities of channels in phospholipids ( Fig. 6c ), and its conductance–voltage curve was right-shifted significantly [33] . These data argue that no high-affinity sites ( k D <75 mM) dictate the lipid–VSD interaction, and that the VSDs are in slow equilibrium between the two lipid-determined conformations because, if the lipid-dependent gating had been a fast process such that four Fv molecules could lock the channel 'up', we should have obtained ~100% Fv-binding. Our observations also explain the weak effects of low %DOTAP and %DOGS on the VSD movement in Fig. 2a . The phosphate–VSD interaction therefore appears to result from multiple low-affinity sites on the VSD that interact with annular lipids. Cholesterol effect on KvAP as predicted by lipid gating Both voltage- and lipid-dependent gating switch the VSDs between two distinct gating conformations ( Fig. 7a ). In membranes of mixed lipids, they probably work together to determine the gating behaviour of the channel. KvAP channels in nature reside in bilayers containing diethers and tetraethers, both C40-based nonphospholipids [49] . They should therefore experience both lipid- and voltage gating, and their gating properties are expected to change when their host bacteria drift from one habitat to another. A prediction from lipid-dependent gating is that natural nonphospholipids including cholesterol, some glycolipids and positively charged lipids, should modulate the VSDs. Indeed, even though a KvAP channel never encounters cholesterol in A. pernix membranes, its voltage-dependent activity was completely lost in well-mixed DOPC (1,2-dioleoyl- sn -glycero-3-phosphocholine) bilayers containing more than 10% cholesterol (weight ratio, ~18% molar ratio; Fig. 7b and Table 2 ) [50] . Cholesterol molecules disturb the packing of lipid head groups as well as the acyl chains in a bilayer [51] . Their hydroxyl head groups presumably partitioned into annular lipids, alienated phospholipids from the VSDs and exerted lipid-gating effects. 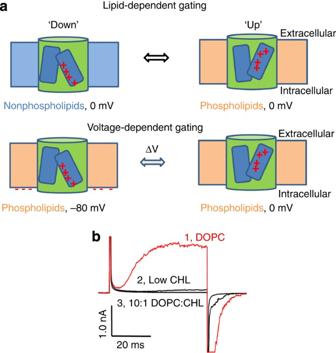Figure 7: Lipid-dependent gating works together with voltage gating in mixed membranes. (a) Comparison of lipid-dependent gating with voltage gating. One VSD is schematically shown to have two mobile parts (blue rectangles) that move against each other in membranes, and is coupled to the pore region (green cylinder). Switching lipids in membranes (blue for nonphospholipids and orange for phospholipids) changes the VSD conformations (lipid-dependent gating, top row) in the same way as the voltage gating (bottom row) does. (b) Lipid-dependent gating and voltage gating work together in a DOPC/cholesterol (CHL) membrane. The KvAP channels function normally in DOPC membranes (red trace1on the left), but behave differently in cholesterol-containing membranes (10:1 DOPC/CHL weight ratio; trace3, typical fromn=28). When channels in DOPC (for trace1) were introduced into membranes for trace3(10:1), the cholesterol concentration was diluted to <10% (the membrane is expected to be in a liquid disordered phase as inTable 2), and small currents (trace2, typical fromn=5) could be recorded. Figure 7: Lipid-dependent gating works together with voltage gating in mixed membranes. ( a ) Comparison of lipid-dependent gating with voltage gating. One VSD is schematically shown to have two mobile parts (blue rectangles) that move against each other in membranes, and is coupled to the pore region (green cylinder). Switching lipids in membranes (blue for nonphospholipids and orange for phospholipids) changes the VSD conformations (lipid-dependent gating, top row) in the same way as the voltage gating (bottom row) does. ( b ) Lipid-dependent gating and voltage gating work together in a DOPC/cholesterol (CHL) membrane. The KvAP channels function normally in DOPC membranes (red trace 1 on the left), but behave differently in cholesterol-containing membranes (10:1 DOPC/CHL weight ratio; trace 3 , typical from n =28). When channels in DOPC (for trace 1 ) were introduced into membranes for trace 3 (10:1), the cholesterol concentration was diluted to <10% (the membrane is expected to be in a liquid disordered phase as in Table 2 ), and small currents (trace 2 , typical from n =5) could be recorded. Full size image Table 2 KvAP activity in DOPC /cholesterol (CHL) mixed bilayers. Full size table Our data on Fv-binding, cysteine accessibility pattern, VSD-pore domain coupling and the selection of cognate peptide ligands exhibited high mutual consistency, and led to two main conclusions. Without any transmembrane potential, lipid-dependent gating switches the VSDs 'up' and 'down', and the pore domain 'open' and 'closed'; the lipid bilayer surrounding the VSDs (annular lipids) is a determining factor for lipid-dependent gating. The majority of these lipids are not among the structural lipids seen in the high-resolution structure of the Kv1.2/2.1 chimera, in which most lipids were ordered in the 'concave hemi-circles' between neighbouring VSDs [22] . The lipid-dependent gating is strong and homogeneous, and its estimated energetic change is close to that of the voltage-dependent gating. The free energy gained through DOTAP–channel interaction (stabilize the 'down' conformation) is higher than 12 kcal mol −1 (valence of 5.0 in a 100 mV step, Fig. 1b ), but should be lower than 60 kcal mol −1 (binding energy of four Fv fragments needed to keep the VSDs 'up' in DOTAP, Fig. 4a and Supplementary Fig. S2 ). This estimate is close to the ~30 kcal mol −1 that is required to relocate 13 elementary charges (in each Shaker -type Kv channel) across a membrane and stabilize the 'down' conformation [7] ( Fig. 7a ). The annular lipids could therefore consume part of the energy input from the gating charge movement, and help to set the energy level at the mid-point potential ( V 1/2 ) of the voltage-dependent VSD movement ( Fig. 2a ). Considering the multiple low-affinity sites for phospholipids (assuming k D ~100 mM), each VSD in one channel needs five to six sites to reach 30 kcal mol −1 . A four-helical VSD is similar in size to one aquaporin-0 monomer [52] . But because the KvAP VSDs presumably contact lipids at three sides, it may have 10–15 annular lipids, enough to contribute the needed interaction sites. The energetic stabilization of the two lipid-determined conformations has to result from both the VSDs and the lipids. Because DOTAP has the same acyl chains as DOPC ( Supplementary Fig. S1 ), the lipid-gating effect must come from lipid head groups: either the absence of the phosphodiesters or the charged trimethyl-ammonium ions in DOTAP being closer to the glycerol backbone than in DOPC. Should it be the positive charges in DOTAP that drove the VSDs to the 'down' conformation, we would not have seen the same effects in negatively charged DOGS membranes. In addition, by electrostatic shielding, 1.0 M free phosphate per 0.45 M KCl in our Fv-binding assays failed to relieve the VSDs from the 'down' state in DOTAP vesicles. It is therefore very likely that the groups replacing the phosphodiesters determine the lipid-dependent conformational switch. What is shared by DOTAP and DOGS is that less polar groups replace the phosphodiesters and do not form as extensive an H-bonding network. It is conceivable that the VSDs in the 'down' conformation better tolerate these groups in DOTAP or DOGS. We propose that the switch of the VSDs from 'down' to 'up' is accompanied by the exposure of more polar residues at the level of two phosphate layers in membranes. This proposal echoes well with the recent observation that higher hydrophobicity at the six positions interposed between the four S4 arginines favours a more stable 'down' conformation of the Shaker VSDs [23] . What is really unique about the two phosphate layers that contributes to the lipid-dependent gating? Molecular dynamics simulation indicated that the phosphate layers could be distorted at the lipid–VSD surface [53] . Electron crystallographic structures of aquaporin-0 in different lipids showed that the distance between two phosphodiester layers in the annular lipids ('phosphate belts') remains roughly the same among membranes with varying lipid composition, and the pattern of the acyl chain/protein interaction (hydrophobic interaction) is well preserved [52] . The discrepancy here may reflect the major differences between the two proteins. Aquaporin-0 functions as a rigid connector between two apposing membranes, whereas the VSD undergoes a major structural rearrangement inside its resident bilayer. Presumably the pattern of phosphate–VSD interaction varies when the VSD switches its conformations, and changing such a pattern of interaction forges the structural basis for lipid-dependent gating. Furthermore, the lipid-dependent gating raises the question whether a VSD could change its conformation when the channel is transferred from detergents or detergent/lipid micelles into a real bilayer, and vice versa . In a more general sense, for membrane proteins that experience strong lipid–protein interaction, it is important to investigate how well detergent micelles or bilayer mimicries support their specific functional states [51] , [54] . The cholesterol effect on the KvAP function is a natural prediction from our working hypothesis ( Fig. 7 ), and offers an explanation to earlier observations that KvAP channels expressed in Xenopus oocytes and in culture cells failed to function (K. Swartz, personal communication), possibly due to high-cholesterol content in the plasma membranes or the expressed channels being delivered to cholesterol-enriched domains. Still the successful expression and delivery of KvAP channels in these cells needs verification. Given the possible high content of C40-based ether lipids in A. pernix membranes, the KvAP channels should be largely suppressed in native cells at room temperature, but could become more active at elevated temperature. For eukaryotic voltage-gated channels, native nonphospholipids in cell membranes come into play. Several groups have studied the effects of cholesterol manipulation on eukaryotic voltage-gated ion channels [30] , [31] , [32] , [45] , [55] . Because none of them could record ionic currents from channels exclusively in cholesterol-enriched microdomains, the observed cholesterol effects by whole-cell recording were much weaker than our observations in homogeneous membranes ( Fig. 7b ), and some even conflicted with each other. It is interesting to note that because of the preferential packing between sphingomyelin and cholesterol [27] , the effects of sphingomyelinase treatment [34] , [35] may be related to the cholesterol effect. It will be very informative to examine a eukaryotic voltage-gated ion channel in DOPC/sphingomyelin/cholesterol ternary membranes. Furthermore, it is worth pointing out that because cholesterol and sphingomyelin are not usually present in prokaryotes, the cholesterol effect could be stronger on prokaryotic channels (including KvAP) than on eukaryotic ones, as the latter might have been evolved to function in cholesterol/sphingomyelin-enriched membranes. Needless to say the cholesterol/sphingomyelin effect will be important for the possible metabolic control of voltage-gated ion channels in vivo . Even though at a first glance our cholesterol data seem to represent direct connections to the co-evolution of lipids and membrane proteins [26] , the co-evolution argument remains uncertain. The concept originated from the lipid-dependent topogenesis observed in some transport proteins [26] . In our experiments, the KvAP and its mutants suffered no topological change. Further, a bacterial voltage-gated sodium channel functioned well in eukaryotic cells [56] , [57] , obviously escaped from the co-evolution prediction and probably delivered to cholesterol-sparse microdomains in these cells. Another clear difference between the lipid-dependent gating and the lipid-dependent topogenesis is on their chemical basis. Lipid-dependent topogenesis seemingly results from head group difference (PE/PC versus PG/cardiolipin) as well as the interplay between translocon, lipids and transmembrane segments [26] . Our lipid-dependent gating apparently results from the low-affinity lipid–protein interactions at the levels of the two phosphate layers. We therefore believe that the conceptual co-evolution of voltage-gated ion channels with their natural lipid membranes awaits more supporting evidence. In conclusion, both lipid- and voltage-dependent gating switch the VSDs between the same two conformations, and exhibit similar energetic requirements. We propose that both the annular lipids and a channel protein are necessary to form a functional voltage-gated ion-conducting unit, and in mixed membranes such as cell membranes that contain both phospholipids and nonphospholipids, lipid-dependent gating and voltage-gating work together to determine the opening or closing of voltage-gated ion channels. Production and reconstitution of the KvAP and its mutants Constructs of wild-type KvAP and KvAPΔ36 were obtained from Dr Roderick MacKinnon's laboratory. The channels and their mutants were produced by following a published procedure [58] . For reconstituting the channel proteins into DOTAP and DOGS, the lipids were prepared differently. DOTAP was sonicated to form vesicles, and 10 mM decyl-maltoside (DM) and 40 mM β-OG (β-octyl-glucoside) were introduced to completely solubilize the vesicles. For DOGS, overnight incubation with 10 mM DM per 60 mM β-OG was used instead. For the mixture of DOGS or DOTAP with phospholipids, the amount of β-OG was adjusted to achieve complete lipid solubilization. Fv and its mutant The cDNA construct for recombinant 33H1 Fv was a generous gift from Dr Roderick MacKinnon's laboratory, and was produced as described previously [36] . Site-specific mutation was introduced using QUICKCHANGE kit. To make a fluorescent Fv, a cysteine residue was introduced at position 61 of the heavy-chain FvA61C. The mutant protein was purified, reduced with 5.0 mM DTT, run through a Superose 12 column (GE Health Science) to remove DTT, mixed with 1.0 mM Alexa 488 maleimide (Invitrogen), and incubated in dark at 4.0 °C overnight. FvA61C-Alexa 488 was purified by Fast Protein Liquid Chromatography (FPLC). Based on the absorption spectra of FvA61C and Alexa 488, the conjugation efficacy was 90–95%. Binding assay of FvA61C-Alexa 488 to channels in vesicles Reconstituted channels were mixed with FvA61C-Alexa 488 (0–200 μg ml −1 ). The mixture was adjusted to 1,000 μl, and spun for 45 min at 250,000 g at 4 °C. The supernatant was discarded, and the tube wall was washed once without disturbing the pellet. The pellet was dissolved in 20 mM DM, and measured at the 537 nm in a Perkin-Elmer LS55 fluorospectrometer (Perkin-Elmer), using a 495 nm excitation beam and 2.5 nm slits. To measure nonspecific binding, the same volume of vesicles was incubated with 400 μg ml −1 unlabelled Fv before FvA61C-Alexa was added. Recombinant CTX and its binding assay The constructs for wild-type CTX and CTXR19C were kindly provided by Dr Christopher Miller (Brandeis University). The production of recombinant CTX followed a published procedure [59] , except that the final purification was achieved in a Resource S FPLC column. For Alexa 488 conjugation, CTXR19C was reduced (5.0 mM DTT) and purified by FPLC before reacting with fivefold molar excess of Alexa 488 maleimide in dark for ~10 h at 4 °C. The conjugates were purified by FPLC. To measure the binding of the CTX-R19C-Alexa 488 to channels in vesicles, a centrifugation procedure similar to that for Fv-A61C-Alexa was used. Fluorescent CTX varied between 0.1 to 5 μM, and 100 μM wild-type CTX was used in control samples to measure nonspecific binding. Vesicle floatation experiment Vesicles (150 μl) were mixed with 150 μl of 30% Ficoll 400 in 100mM KCl, 20 mM HEPES-KOH pH 7.4, and loaded into a 1.2 ml centrifuge tube; 400 μl 10 and 0% Ficoll 400 solutions were laid afterwards. The gradient was spun at 250,000 g , 4.0 °C, 2 h. Fractions (~140 μl) were collected from top to bottom for SDS–PAGE. Channels in phospholipids were found at 10–15% interface, and those in DOTAP or DOGS at 0–10% interface ( Supplementary Fig. S4 ). Gel-shift assay of KvAP cys-mutants by MTSPEG5k Reconstituted KvAP cysteine mutants were reduced with 5.0 mM DTT at room temperature for 30 min, pelleted down by spinning at 250,000 g , 4 °C, 45 min, washed twice with DTT-free buffer and reacted with 1.0 or 2.0 mM MTSPEG5k for 30 min. The reaction was stopped with 10 mM iodoacetamide (Sigma). DM (20 mM) was added before nonreducing SDS–PAGE. Screening for tight binders to KvAP in DOTAP/DOGS vesicles A phage-displayed 20mer peptide library was kindly provided by Dr. Kathlynn Brown [60] . Peptides were at the amino termini of the pIII protein in the filamentous bacteriophage fd-tet. The library contains 1.0×10 8 random sequences. Panning, titering and amplification of the phages followed the established procedures in the Brown laboratory. For biopanning, channel vesicles supplemented with 0.10% biotinylated POPE (Avanti Polar lipids) were pulled down with neutravidin-coated beads (Pierce). Supplementary Figure S6 showed a general flowchart. After 14 runs, positive colonies were selected for PCR and sequencing. Four positive clones (A–D) were identified, and clones B and D showed much stronger effects on KvAP. Synthetic peptide of clone D (φ D ) was prepared in the protein core laboratory at the UT Southwestern Medical Center, and was purified as a single peak in a C18 HPLC column (>99% purity). Its molecular weight was verified by mass-spectroscopy. To test the effect of φ D peptide on KvAPΔ36L125C in PE/PG membranes, reduced channels in vesicles were divided into two halves: one as control and the other with 100 μM peptides for 5 min. Later steps were the same as in Figure 4a . The peptide effect on KvAP T225C in PE/PG was tested differently from Figure 4c , because the peptide does not cross the membranes. Reconstituted channels were treated with 5.0 mM DTT and 100 μM peptide, separated from DTT, resuspended with DTT-free peptide-rich buffer containing 5.0 mM GSSG, and after 2–3 min analysed by nonreducing SDS–PAGE. Electrical recordings from channels in lipid bilayers A tabletop vibration isolation system (Warner Instruments) was purchased to support the bilayer recording chamber inside a Faraday cage. A gravity-driven perfusion system was used to introduce 15 ml of solution to either side of the bilayer per minute. A total volume of 20 mg ml −1 lipids in decane [33] were used to paint a bilayer across a 150 or 200 μm hole in a recording cup. An Axopatch 200B patch-clamp system in the whole-cell voltage-clamp mode recorded ionic currents. Once a membrane was stable, a small volume (0.4–1.0 μl) of channel vesicles was injected onto it. Every 2 min a test pulse from a holding potential of −80 mV to +80 mV for 100 ms was delivered. The inactivation suppressed channels facing the opposite directions at holding potentials. All reported current traces followed the electrophysiological convention that outward currents go upwards. How to cite this article: Zheng, H. et al . Lipid-dependent gating of a voltage-gated potassium channel. Nat. Commun. 2:250 doi: 10.1038/ncomms1254 (2011).